Winter and spring controls on the summer food web of the coastal West Antarctic Peninsula Understanding the mechanisms by which climate variability affects multiple trophic levels in food webs is essential for determining ecosystem responses to climate change. Here we use over two decades of data collected by the Palmer Long Term Ecological Research program (PAL-LTER) to determine how large-scale climate and local physical forcing affect phytoplankton, zooplankton and an apex predator along the West Antarctic Peninsula (WAP). We show that positive anomalies in chlorophyll- a (chl- a ) at Palmer Station, occurring every 4–6 years, are constrained by physical processes in the preceding winter/spring and a negative phase of the Southern Annular Mode (SAM). Favorable conditions for phytoplankton included increased winter ice extent and duration, reduced spring/summer winds, and increased water column stability via enhanced salinity-driven density gradients. Years of positive chl- a anomalies are associated with the initiation of a robust krill cohort the following summer, which is evident in Adélie penguin diets, thus demonstrating tight trophic coupling. Projected climate change in this region may have a significant, negative impact on phytoplankton biomass, krill recruitment and upper trophic level predators in this coastal Antarctic ecosystem. The western continental shelf region of the West Antarctic Peninsula (WAP) is experiencing rapid climate change [1] and one of the fastest rates of winter warming on Earth [2] . Associated changes include significantly reduced sea ice extent, concentration and duration [3] , [4] , and accelerated retreat and melting of glaciers and ice sheets [5] , [6] . As life histories of most polar organisms are attuned to ice seasonality, recent warming and declines in sea ice have been associated with changes at key trophic levels in the food web of the WAP region north of Palmer Station, including a reduction in phytoplankton biomass [7] , shift in phytoplankton community composition from large diatoms to small flagellated cryptophytes [7] and reduction in the abundance of Antarctic krill ( Euphausia superba ; determined from data sets spanning mid-1970s to 2003) (refs 8 , 9 ). In addition, a decline in Adélie penguins ( Pygoscelis adeliae ) near Palmer Station has occurred over the past three decades [10] . Krill are the main trophic link between phytoplankton and many apex predators in Antarctic food webs [9] , [11] . Adélie penguin diets in the Palmer region during the past two decades almost exclusively consist of Antarctic krill [12] . Thus, changes in krill abundance and size distribution impact Adélie penguin foraging ecology, specifically their foraging effort (that is, foraging trip duration) [12] . Krill abundance tends to increase following years of good recruitment (high biomass of smaller, younger individuals), and conversely, decrease following years of poor recruitment [12] . Consequently, Adélie penguin foraging trip duration is shortest when krill are most abundant after high recruitment years and longest after poor recruitment years [12] . During long foraging trips, penguins have to use a portion of the gathered food for self-maintenance, resulting in the delivery of less food to their chicks [13] . Thus, one implication of longer foraging trips is that they would have a negative impact on the reproductive output of Adélie penguins and potentially other krill consumers such as Antarctic fur seals, macaroni and gentoo penguins, and albatrosses [12] , [14] . The reported krill decline in the far northern WAP region [8] , [9] is one of many factors suggested to be associated with recent concomitant declines in the Adélie penguin population [15] . In addition to long-term changes, the WAP ecosystem is characterized by high interannual variability [16] , [17] . Phytoplankton dynamics have previously been associated with ice-mediated changes in water column stability [18] , [19] . In turn, sea ice changes are governed by fluctuations in the Southern Annular Mode (SAM) and/or the El Niño-Southern Oscillation (ENSO) [20] , [21] , [22] . Krill recruitment variability has also been linked to sea ice [8] , [12] . In the far northern WAP region near the South Shetland–Elephant Island area, phytoplankton biomass and krill recruitment were regulated by ENSO-driven variability of the location of the southern frontal systems of the Antarctic Circumpolar Current [17] . Interpreting this cascade of changes in the ecosystem requires understanding of the mechanisms linking the physical and biological systems, and the degree of coupling between them. Using data collected since 1991 from the Palmer Long Term Ecological Research program (PAL-LTER) Stations B and E near Palmer Station ( Supplementary Fig. 1 ), we provide the first multi-decadal analysis from this region and illustrate the succession of large-scale and local physical forcing through trophic levels, from bacteria and phytoplankton to an apex predator. Interannual variability in phytoplankton and bacteria During the 21-year-long PAL-LTER time series (1991–2012), peaks in depth-integrated (0–50 m) summer (December–January–February) chlorophyll- a (chl- a ) concentration at coastal PAL-LTER Stations B and E ( Supplementary Fig. 1 ) have occurred, on average, every 4–6 years ( Fig. 1a ). Although the bacterial productivity (BP) data set is limited to the last decade (2002–2012), the variability in the anomalies follows those of chl- a ( Fig. 1a ), likely because phytoplankton in Antarctic waters provide the main source of dissolved organic carbon for bacterial growth [23] . The two dominant phytoplankton groups in the region are diatoms and cryptophytes (as determined by accessory pigment analysis, see Methods section). The phytoplankton composition during these peak chl- a years was dominated by diatoms, whereas the proportion of cryptophytes increased in anomalously low chl- a years (one-way analysis of variance, P <0.001). Large diatoms (>20 μm) are the preferred prey of krill because krill cannot efficiently feed on phytoplankton <20 μm in diameter [24] . 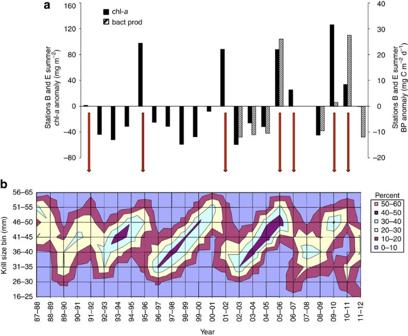Figure 1: Interannual variability of multiple trophic levels of the Palmer Station food web and linkages between them. (a) Summer (December–January–February) depth-integrated (0–50 m) chlorophyll-a(chl-a) and bacterial productivity (BP) anomalies pooled from Palmer Stations B and E for the PAL-LTER time series, 1991–2012 (see Methods section). The average combined (Stations B and E) depth-integrated chl-aand BP for the time series is 108 mg m−2and 32.4 mg C m−2d−1, respectively. (b) Size-class distribution (percent contribution (colours; see legend) of each krill size bin (yaxis)) of Antarctic krill,E. superba, in Adélie penguin diet samples, 1988–2012; modified with permission from Ducklowet al.25The vertical red arrows indicate the appearance of strong new krill cohorts in years following positive chl-aanomalies. Figure 1: Interannual variability of multiple trophic levels of the Palmer Station food web and linkages between them. ( a ) Summer (December–January–February) depth-integrated (0–50 m) chlorophyll- a (chl- a ) and bacterial productivity (BP) anomalies pooled from Palmer Stations B and E for the PAL-LTER time series, 1991–2012 (see Methods section). The average combined (Stations B and E) depth-integrated chl- a and BP for the time series is 108 mg m −2 and 32.4 mg C m −2 d −1 , respectively. ( b ) Size-class distribution (percent contribution (colours; see legend) of each krill size bin ( y axis)) of Antarctic krill, E. superba , in Adélie penguin diet samples, 1988–2012; modified with permission from Ducklow et al . 25 The vertical red arrows indicate the appearance of strong new krill cohorts in years following positive chl- a anomalies. Full size image Link between phytoplankton biomass and krill recruitment Positive chl- a anomalies corresponded to statistically significant krill recruitment events (evidenced in Adélie penguin diet samples), which resulted in the start of a new krill cohort the following season ( Fig. 1b ). This trend is substantiated by significant positive linear trends in summer chl- a with a 1-year lag of R 1 , the recruitment of krill age class year 1+ (percent contribution of krill <30 mm to the total number of krill) ( Fig. 2 ). This suggests that high food availability facilitates increased krill recruitment success by maximizing krill spawning potential (that is, longer spawning season, larger number of eggs per batch, larger number of egg batches, and/or higher egg hatching success) or by supporting higher post-hatching survival and growth rates—the specific responses are not yet known. Thus, food availability (positive chl- a anomalies) appears critical for the success of krill recruitment. In addition, sea ice is crucial for the overwinter survival of younger krill age classes, and specifically the provision of food and refugia from predators for larval krill (overwintering of the year 1+ age class) [8] , [9] , [12] . Hence, krill recruitment is a two-step process in which female condition is improved through high chl- a during summer, and the larval survival is enhanced by high ice cover the following winter [8] , [12] . 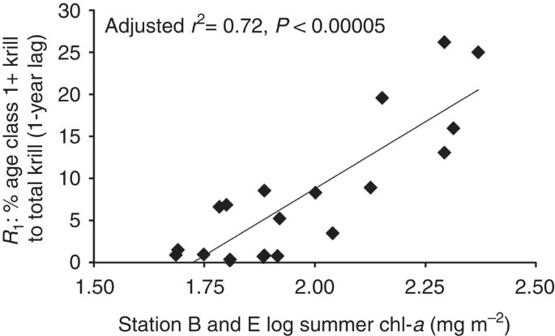Figure 2: Relationship between Palmer Station summer chl-aand krill recruitment. Log-transformed summer (December–January–February) depth-integrated (0–50 m) chlorophyll-a(chl-a) pooled from Palmer Stations B and E (xaxis) versusR1(the recruitment of krill age class 1+, defined as the percent contribution of krill <30 mm to the total number of krill in Adélie penguin diets during each summer; see Methods section) with a 1-year time lag following summer chl-a(n=19, Pearson’sR=0.84, adjustedr2=0.72,P<0.00005). Figure 2: Relationship between Palmer Station summer chl- a and krill recruitment. Log-transformed summer (December–January–February) depth-integrated (0–50 m) chlorophyll- a (chl- a ) pooled from Palmer Stations B and E ( x axis) versus R 1 (the recruitment of krill age class 1+, defined as the percent contribution of krill <30 mm to the total number of krill in Adélie penguin diets during each summer; see Methods section) with a 1-year time lag following summer chl- a ( n =19, Pearson’s R =0.84, adjusted r 2 =0.72, P <0.00005). Full size image Large-scale climate and local physical drivers of chlorophyll From the investigation of potential large-scale and local controls on the cyclical pattern of phytoplankton chl- a variability, we identified both winter and spring controls that act to regulate summer chl- a concentration ( Figs 3 and 4 ). We conducted a stepwise regression analysis to determine how well various combinations of identified local (that is, wind, water column stability, sea ice) and large-scale (that is, SAM; Multivariate ENSO Index, MEI) physical forcing could predict variations in depth-integrated chl- a for each summer. Based on a stepwise regression and model ranking criteria, the highest-ranking models for both Stations B and E log summer chl- a were linear functions. For Stations B and E, physical forcing accounted for 66% and 54% of summer depth-integrated chl- a variability, respectively (Station B: adjusted r 2 =0.66; F-statistic versus constant model, 9.62, P <0.000005; root mean square error=0.149; Fig. 3a . Station E: adjusted r 2 =0.54; F-statistic versus constant model, 7.08, P <0.00001; root mean square error=0.147; Fig. 3b ). The predictor variables of summer chl- a were WAP August ice extent, spring SAM (September–October–November), seasonal (October–February) wind speed, wind speed threshold (number of days per season when wind speed was below 2.5 m s −1 ), November–December stratification and the interactions between these variables. The MEI was not a statistically significant predictor for chl- a . WAP August ice extent was inversely correlated with SAM in July (Pearson’s R =−0.61, P <0.005). The stratification index that most significantly predicted chl- a in the models was Δsigma-theta T min−0 (kg m −3 m −1 ), defined as the density at the temperature minimum ( T min ) in the remnant Winter Water layer (underlying the surface waters) minus the density at the surface. In this region, Δsigma-theta T min−0 is driven primarily by the salinity gradient in the upper water column, and is most pronounced during surface freshening from sea ice melt and retreat in the spring. The interaction between wind threshold and Δsigma-theta T min−0 was the strongest predictor for Station B chl- a ( t -statistic=4.99, P <0.00005), whereas the interaction between WAP August ice extent and wind threshold was the strongest predictor for Station E chl- a ( t -statistic=4.36, P <0.0005); refer to Methods section and Supplementary Tables 1 and 2 for details on the model equations and statistics. These model results indicate that phytoplankton biomass, and indirectly BP, krill recruitment, and Adélie penguin diet composition near Palmer Station, are driven by water column stability, which is influenced by both winter (July SAM, sea ice extent) and spring (SAM, wind, Δsigma-theta T min−0 ) processes. We refer to this preconditioning as the ‘setup event’. Favourable conditions for phytoplankton, specifically diatoms, included increased winter ice extent and duration, reduced spring/summer winds and increased water column stability via enhanced salinity-driven density gradients. 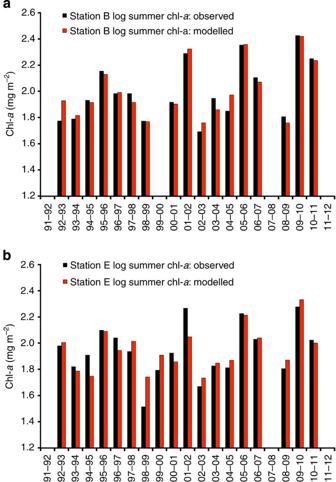Figure 3: Observed versus modelled time series of chl-aat Palmer Stations B and E. A stepwise regression of General Linear Models (GLMs) combined with model ranking criteria identified the predictor variables and their interactions that constrain the average log-transformed summer (December–January–February) depth-integrated (0–50 m) phytoplankton biomass at Palmer Station B (a; Pearson’sR=0.96, adjustedr2=0.67) and E (b; Pearson’sR=0.86, adjustedr2=0.54) in each summer. (See text andSupplementary Tables 1 and 2for details on the model equations, predictors and statistics.) Figure 3: Observed versus modelled time series of chl- a at Palmer Stations B and E. A stepwise regression of General Linear Models (GLMs) combined with model ranking criteria identified the predictor variables and their interactions that constrain the average log-transformed summer (December–January–February) depth-integrated (0–50 m) phytoplankton biomass at Palmer Station B ( a ; Pearson’s R =0.96, adjusted r 2 =0.67) and E ( b ; Pearson’s R =0.86, adjusted r 2 =0.54) in each summer. (See text and Supplementary Tables 1 and 2 for details on the model equations, predictors and statistics.) 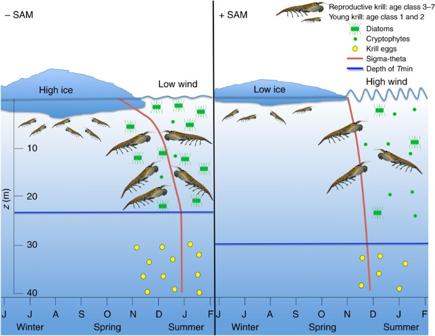Figure 4: Effects of large-scale climate and local physical forcing on biological processes in the coastal WAP. Generalized illustration summarizing how individual and combined winter and spring climate, weather and physical oceanographic processes (see months July–February onxaxis) cascade from phytoplankton to krill recruitment in a negative Southern Annular Mode (−SAM) in July and spring (left panel) and a positive SAM (+SAM) in July and spring (right panel). Depth of temperature minimum (Tmin) in the remnant Winter Water layer in the region was estimated from Stations B and E November–December averages. All other properties (phytoplankton, krill, krill eggs and sigma-theta) are generalized for qualitative illustration (more versus less), and do not represent quantitative differences between negative and positive SAM. Note: femaleE. superbaspawn over deeper water; this illustration is meant to depict relative egg production. Full size image Figure 4: Effects of large-scale climate and local physical forcing on biological processes in the coastal WAP. Generalized illustration summarizing how individual and combined winter and spring climate, weather and physical oceanographic processes (see months July–February on x axis) cascade from phytoplankton to krill recruitment in a negative Southern Annular Mode (−SAM) in July and spring (left panel) and a positive SAM (+SAM) in July and spring (right panel). Depth of temperature minimum ( T min ) in the remnant Winter Water layer in the region was estimated from Stations B and E November–December averages. All other properties (phytoplankton, krill, krill eggs and sigma-theta) are generalized for qualitative illustration (more versus less), and do not represent quantitative differences between negative and positive SAM. Note: female E. superba spawn over deeper water; this illustration is meant to depict relative egg production. Full size image Favourable conditions for phytoplankton growth and krill recruitment typically occurred during a −SAM in winter and spring. SAM variability is characterized by the opposing atmospheric pressure anomalies between Antarctica and mid-latitudes, and is reflected in the strength of subpolar westerly winds [20] , [26] . When SAM is positive (+SAM), warmer north-westerly winds move over the WAP region. The increasing trend of +SAM occurrences has contributed to Antarctic warming trends over the recent decades [27] , [28] . During a −SAM in winter (that is, July), cold southerly winds move across the Peninsula, increasing winter ice extent and duration and delaying ice retreat in spring. Wind speeds and the number of windy days are significantly reduced during a −SAM in spring/summer (October–February, Pearson’s R , P <0.005). The intensity of the local atmospheric response to SAM is also related to ENSO-SAM interactions [22] , [29] , [30] , [31] . Previous studies have shown an intensified atmospheric response (and thus sea ice as well) when a +SAM/La Niña or −SAM/El Niño are coincident (for example, a −SAM coincident with El Niño can amplify blocking high conditions favourable for high winter sea ice and/or late spring retreat), relative to the response when +SAM or −SAM occurs when ENSO is otherwise neutral, and vice versa [22] , [30] , [31] . Conversely, a dampened response occurs when +SAM/El Niño or −SAM/La Niña were coincident. Thus, although the results in the current study indicate that SAM is a significantly stronger predictor of chl- a (due to direct, regionalized influence on winds, ice, water column stability and so on) compared with ENSO (MEI), the concurrent influence from SAM/ENSO interactions is embedded in the SAM index time series. Both increased winter sea ice (extent and duration) and reduced winds in spring–summer contribute to the increase in salinity-driven density gradients (Δsigma-theta T min−0 ) in the upper water column. Whereas individual factors of winter and spring forcing can constrain seasonal phytoplankton dynamics, the combined interactions between these factors, as dictated by SAM, drive the overall summer biological processes ( Figs 3 and 4 ). Relatively, high ice extent in the winter likely facilitates higher stratification in the following spring and summer via two mechanisms: first, by insulating the water column from high winter winds and thus preventing the formation of a deep winter mixed layer [7] , [19] ; and second, by providing a larger volume of sea ice melt water that strengthens the density gradient in the upper water column in the following spring and summer [18] . Similar to Marguerite Bay farther south along the WAP [19] , Palmer November–December mixed layer depth (MLD) was not significantly correlated with summer chl- a . However, the depth of November–December T min (that is, the Winter Water core) was on average ~\n8 m shallower during years with higher chl- a (one-way analysis of variance, P <0.05; Fig. 4 ). Stratification indices Δsigma-theta T min−0 and MLD were also associated with the timing of sea ice retreat (Pearson’s R =0.70 and P <0.005 for MLD; Pearson's R=0.50 and P <0.05 for Δsigma-theta T min−0 ), suggesting that later sea ice retreat in the spring may provide additional wind protection and assist in maintaining water column stability. Similar mechanisms were suggested for Marguerite Bay, farther south along the WAP, in which years with longer winter ice cover favoured larger summer blooms as a consequence of a shallower winter mixed layer, resulting in greater water column stability the following summer [19] . During light ice cover winters, the winter mixed layer was deeper, and water column stability and chl -a content were lower the following summer [19] . There were no statistically significant correlations between chl- a and cloud cover or surface macronutrient concentrations (macronutrients are seldom depleted in the WAP region [10] ). Long-term dissolved iron data were not available for this region. Venables et al . [19] argue that increased stratification promotes phytoplankton growth via reducing the variability in light conditions (as opposed to enhancing overall light availability), and may concentrate iron from glacial melt water inputs in the upper water column. Therefore, the mechanisms driving the dynamic relationship between water column stability and phytoplankton biomass could be light and/or iron limitation and need to be investigated further. Similarly, the roles of sea ice loss, ocean freshening, light and nutrient limitation on Arctic Ocean marine primary productivity also remain poorly understood, with some studies indicating shifts from larger nanoplankton to smaller picoplankton dominance owing to enhanced stratification from increased river runoff [32] , [33] , [34] . One current paradigm regarding the origins or ‘source’ populations of krill in the WAP invokes the transportation of larvae ‘upstream’ from the Bellingshausen Sea in the southwest to the coastal shelves in the northeast via the Antarctic Circumpolar Current [35] , [36] . However, the occurrence of very small krill (≤16 mm) present in Adélie penguin diets in our study area [12] ( Fig. 1b ) has led to suggestions that certain areas of the WAP including the Palmer Station region are indicative of a more localized, self-sustaining krill population [12] , [37] . Furthermore, previous studies identified the Palmer Station region (Anvers Island) as a retention area, where larvae spawned from adult krill likely remain in the region and sustain a local krill population [37] , [38] . The tight linkages demonstrated between local physical forcing and phytoplankton and krill in our study also support the idea that localized processes may be more important than remote ‘upstream’ processes in forcing the system in the Palmer Station region. Changes in the WAP climate and ecosystem have been profound over the past 50 years [1] , and include significant declines in sea ice [3] , [4] , phytoplankton biomass [7] and krill [8] , [9] in the region north of Palmer Station. Global climate model projections under continued greenhouse gas emission scenarios up to the year 2100 suggest a further increase in temperature [39] and an increase in the occurrence of +SAM [20] , [27] , [40] . Repercussions of this projection are the continued increase in the strength of warm, north-westerly winds [21] and decline in sea ice [4] , which will act to reduce water column stability. We hypothesize that this trend will migrate south along the WAP in the next few decades and perhaps expand to other Antarctic regions undergoing a long-term decline in sea ice. Fewer preconditioning ‘setup events’ will act to decrease phytoplankton biomass, favourable krill prey (diatoms) and krill recruitment. Interestingly, our analysis of E. superba abundance in the full PAL-LTER sampling region (Palmer Station and southward) over the last two decades shows no overall long-term decline (in contrast to declines previously documented north of Palmer Station [8] , [9] ), but rather shows abundance peaks (positive anomalies) occurring every 4–6 years. Antarctic krill age class structure is dominated by single, strong cohorts [12] , which we show to be highly dependent on summer phytoplankton biomass in this coastal site. Currently, chl- a anomalies occur every 4–6 years and are associated with −SAM. The Antarctic krill lifespan ranges 6–7 years, which is in the range of the current 4–6 year cycle in positive chl- a anomalies. Thus, an increase in the occurrence of +SAM resulting in even one cycle being longer than the krill lifespan could be catastrophic to the krill population. A recent sensitivity analysis suggests that a decline in summer chlorophyll concentration could have more significant impacts on Antarctic krill biomass than direct effects of warming [41] . A decline in Antarctic krill will negatively impact higher trophic levels dependent on Antarctic krill including penguins, flighted sea birds, seals and whales, most notably their foraging effort and reproductive output. Seawater sampling The PAL-LTER program has been sampling in the Palmer Station region (64.8°S, 64.1°W) in the austral spring-fall annually since December 1991. We examined data from December 1991 through February 2012. The main sampling locations at Palmer Station are an inshore station B (depth ≈75 m) and a more offshore Station E (depth ≈200 m; Supplementary Fig. 1 ), both within the Adélie penguin foraging area. Sampling at each station is conducted via Zodiac, whereby a Conductivity, Temperature, Depth sensor (CTD) is lowered manually for a vertical profile of water column physics, immediately followed by a Go-Flo bottle cast to collect seawater at selected depths for standing stock and rate measurements (that is, chlorophyll, phytoplankton pigments, primary productivity and BP). Seawater from each depth is stored in dark amber Nalgene bottles and processed immediately upon returning to the laboratory at Palmer Station. The goal of PAL-LTER is to sample Stations B and E twice per week from mid-/end of October to mid-/end March. However, successful sampling in this region is heavily dependent on weather, sea ice, time and personnel. Thus, data gaps exist for this time series, whereby some seasons, specifically those early in the time series, had limited or irregular sampling. Data exist for all years except 2007–08. Nonetheless, the summer months of December, January and February (DJF) were the most consistently sampled consecutive months. When data were available for the full sampling season (October–March), the depth-integrated mean chl- a during DJF was almost always higher than when all months (October–March) were pooled together, suggesting that maximum phytoplankton biomass typically accumulated in summer. Thus, we considered DJF a sound representation of the biological growing season and we used these months to estimate summer averages of biological data. Because we believe local physical and large-scale climate drivers create a ‘setup event’ regulating phytoplankton growth, we examined data in the months before the DJF summer maximum. Monthly sample sizes for each measured property are summarized in Supplementary Table 3 . All raw data collected by PAL-LTER (chlorophyll, accessory pigments, BP, physical oceanographic data and penguin diet composition) are available at: http://oceaninformatics.ucsd.edu/datazoo/data/pallter/datasets . Other data, including sea ice properties, meteorological and climate indices had no data gaps during the time period examined. Chl- a and accessory pigments Seawater collected from Go-Flo bottles at different depths was filtered onto GF/F filters, then the filters were wrapped in foil and frozen at −80 °C for fluorometric phytoplankton chl- a analysis [42] (mg chl- a m −3 ); or flash frozen in liquid nitrogen and stored at −80 °C for high-performance liquid chromatography analysis for phytoplankton accessory pigments/phytoplankton composition [43] (mg pigment m −3 ). The taxonomic composition of the phytoplankton assemblages was derived quantitatively from an analysis of high-performance liquid chromatography pigment data with CHEMTAX (V195) (refs 43 , 44 ) using initial pigment ratios previously derived from WAP phytoplankton [45] . For each vertical profile, we calculated the depth-integrated chl- a and accessory pigments (0–50 m; mg m −2 ). The two dominant algal groups in the region are diatoms and cryptophytes. On average prymnesiophytes, prasinophytes and mixed flagellates account for <20%, 5% and 5% of the chl- a biomass, respectively. Sampling in five seasons (1993/1994, 1994/1995, 2001/2002, 2003/2004 and 2004/2005) had few vertical profiles that extended to 50 m. For these profiles, we integrated to the deepest depth sampled (median=40 m); thus, depth-integrated chl- a was likely slightly underestimated. As mentioned above, data gaps exist in the biological data, specifically for early (October and November) and late (March and April) months. Thus, seasonal (summer) chl- a averages were calculated using only DJF data. The chl- a at Stations B and E did not differ significantly in magnitude or variability over time; thus, chl- a data for these two stations were combined then averaged. The average combined depth-integrated summer (DJF) chl- a for the analysed 21-year time series (1991/1992–2011/2012 season) was 108 mg m −2 . Anomalies for each season were calculated from this average and plotted in Fig. 1a . Bacterial productivity Bacterial measurements commenced at Palmer Station in the 2002/2003 season. BP was not measured during the 2006–2007 and 2007–2008 seasons. All measurements are from the same samples as the chl- a data and are similarly integrated to 50 m. BP (mg C m −2 d −1 ) is estimated from the rate of 3H-leucine incorporation measured in 3–6 h incubations performed in the laboratory at Palmer Station in the dark at in situ temperatures [46] . BP was converted from leucine incorporation rates using the factor 1,500 g C biomass produced per mole leucine incorporated. Data were combined and averaged as for chl- a . Water column stability/stratification parameters Over the course of the programme, physical oceanographic data (temperature and conductivity as a function of pressure) were collected using several instruments. From 1991 to 2007, a SeaBird Elecronics ( www.seabird.com ) Seacat SBE 19 was used. From 2006 onwards, a SeaBird Elecronics Seacat SBE 19plus was used, except in field season 2008–2009 (see below). We accounted for sensor drift using calibrations made before and after each field season, following methods recommended by SeaBird, assuming linear drift for well-behaved sensors. We used SeaBird’s standard software functions to process the data, removing effects for zodiac heave (pressure reversals), and to ensure that the temperature, conductivity and pressure were measured on the same water parcel. Data were averaged into 2 db pressure bins for the older SBE 19 data and 1 db bins for the newer instrument, which samples at twice the frequency. Conductivity data were then converted to salinity. From 2008 on, a Falmouth Scientific Inc. FSI MCTD-3 and a Satlantic HyperPro-II (which includes temperature, conductivity and pressure ancillary sensors) were also used to collect physical oceanographic data. As much as possible, we followed the same methods to process these data. The three instruments combined provided full data coverage every time water samples were collected. Plots of each cast were inspected visually and in relation to other casts to look for any issues with the data (for example, bad surface values due to sea state). These values were removed from the data set. Sigma-theta (density; kg m −3 ) was calculated for each pressure bin. A temperature minimum ( T min ) and its depth (in metres) were determined for each cast, ensuring that they represented the remnant cold Winter Water from the previous winter and thus have some warmer water below. The sigma-theta gradient to T min (Δsigma-theta T min−0 ; kg m −3 m −1 ) is defined as sigma-theta at the depth of T min minus sigma-theta at the surface divided by the depth difference between the two. The mixed layer depth (MLD; in metres) is defined as the deepest point of the well-mixed layer of water at the surface, above T min . The method looks for the strongest (weighted) inflection point in temperature (towards colder temperatures and above T min )—further details may be found in Martinson and Iannuzzi [47] . It is thus warmer and less salty than waters below it. We used November–December averages of the stratification indices (depth of T min , Δsigma-theta T min−0 , MLD) from each season for this analysis as this was the time period the data were most significantly correlated to summer chl-a. Adélie penguin diets and krill population size-class structure Adélie penguin diet samples were obtained during January–February for the years 1988 (1987–1988 field season) to 2012 (2011–2012 field season) from adult penguins during the chick-feeding phase of the reproductive cycle. Samples were obtained by using the water off-loading method (forced regurgitation through stomach lavage [48] ), and birds were released unharmed after sampling. All wildlife handling methods were reviewed and approved by the Institutional Animal Care and Use Committee at Marine Biological Laboratory, Woods Hole, MA, USA, protocol suite no. 11–67. Typically, 4–5 Adélie penguins were sampled at 5–7-day intervals during the field season. Following sorting of the diet samples, ingested krill were measured from the base of the eye to the tip of the telson and assigned to 1 of 8 size categories (5 mm increments) between 16 and 65 mm. Because krill grow >5 mm per year [49] , this binning resolves changes in population size-class structure that occur between years. Only whole, fresh krill originating from the upper portion of the stomach were measured. These typically are the first to be off-loaded and their fresh state clearly separates them from the more digested layers that often follow. In all cases, the krill measured represented a subsample obtained by sorting through the entire fresh sample to ensure that smaller specimens were not overlooked; 50–100 krill were typically measured in each subsample. The recruitment index ( R 1 ) is based on the relative abundance of the l+ age class (the ratio of the number of krill aged 1 year to the number of total krill). We defined our 1+ age class as krill <30 mm in length. Because the krill length data are assigned to bins in 5 mm increments, this size group is just above the 1+ age class used in most previous studies (krill <28 mm (refs 50 , 51 , 52 )). However, recruitment years have been estimated with similar distributions using krill <36 mm (ref. 53 ). The R 1 data were normally distributed (Jarque–Bera [54] and χ 2 -tests, P <0.05). Sea birds are good proxy indicators of the spatial and temporal variance associated with the structure (length–frequency distribution) of their prey populations [12] , [55] , [56] . Net tows have not been collected at the local Palmer Station sites (including Stations B and E) owing to lack of appropriate equipment (that is, no winches on small boats). Net tows have been conducted during the January LTER offshore cruise since 1993. We are most confident of the more recent size-class data. Starting in January 2009, the abundance tows were split evenly with all the krill in a split portion measured for size. Thus, we believe that the krill size-class net tow data from 2009 onwards is a close representation of the overall krill population. We compared net tow data from the LTER cruise 600 line, which includes cruise sampling stations closest to Palmer Station ( Supplementary Fig. 2 ), with Adélie penguin diet data from 2009 onwards ( Supplementary Fig. 3 ). The two data sets are in good agreement (2009–2012 combined; Pearson’s R =0.86, adjusted r 2 =0.74, P <0.000001), demonstrating that size-class data collected from Adélie penguin diets are a good representation of the overall krill population in this region. Climate indices Monthly SAM data were obtained from the National Environment Research Council—British Antarctic Survey [26] ( http://www.nerc-bas.ac.uk/icd/gjma/sam.html ). Monthly MEI was obtained for the length of the PAL-LTER time series from National Oceanic and Atmospheric Administration, Earth System Research Laboratory, Physical Sciences Division [57] ( http://www.esrl.noaa.gov/psd/data/correlation/mei.data ). Both SAM and MEI climate indices were tested for correlations with physical (sea ice, air temperature, sea surface temperature (SST) and wind) and biological (that is, chlorophyll) properties assuming no lag and various lag times (1–6 months). SAM was statistically a better predictor than MEI for physical properties (WAP August ice extent, wind, Δsigma-theta T min−0 ) and chl- a . Sea ice WAP (~\n60°–80°W) monthly and Anvers (within 200 km south and west of 64S/64W) annual sea ice extent (km 2 ) and area (km 2 ) were extracted from the GSFC Bootstrap SMMR-SSM/I Version 2 quasi-daily time series (1991–2012) of sea ice concentration [58] from the EOS Distributed Active Archive Center at the National Snow and Ice Data Center (University of Colorado at Boulder, http://nsidc.org ), augmented with SSM/I and near real-time data (2011–2012), to produce a time series extending from 1991/92 to 2011/12. Sea ice extent is defined as the total area within the ice edge, whereas sea ice area is the actual ocean area covered by sea ice (that is, based on satellite-derived sea ice concentration and taking into account openings and leads within the ice edge). Anvers annual ice season duration is the number of days between when sea ice first appears in autumn in a given location and when it last appears in spring, the former being the day of sea ice advance, the latter, day of sea ice retreat [22] . Wind and air temperature Daily weather observations (air temperature, pressure, wind speed, wind direction, precipitation and sky cover) at Palmer Station, Antarctica started in April of 1989. Weather data acquisition was originally by manual observation and continued with an automated system installed in November 2001. Measurements began shifting from manual to automated observations in June 2003 until the manual observations were ended in December 2003. Data are collected, compiled and distributed by the US Antarctic science support contractor. Electronic distribution occurs monthly from Palmer Station via internet to the University of Wisconsin-Madison’s Antarctic Meteorological Research Center and Automatic Weather Station Project archive: ftp://amrc.ssec.wisc.edu/pub/palmer/climatology/ . Data are also available at: http://oceaninformatics.ucsd.edu/datazoo/data/pallter/datasets . Wind speeds were averaged monthly and seasonally (October–February). The PAL-LTER time series average wind speed for October–February was 4.8 m s −1 . Because a potential mechanism to set up water column stability is a time period of low winds, we also calculated the number of days per season (and number days per month) of wind speeds under 4.8 m s −1 , as well as the maximum number of consecutive days under 4.8 m s −1 per season (and per month). We tested additional wind thresholds, and 2.5 m s −1 was most significantly correlated with Δsigma-theta T min−0 and chl- a . Air temperature data was processed (seasonal and monthly averages) similar to wind data. Sea surface temperature Monthly SST data (°C) used in this study originated from the National Oceanic and Atmospheric Administration, National Centers for Environmental Prediction, Environmental Modeling Center, Climate Modeling Branch, Global monthly SST data [59] (version 2). The selected data were SST estimates from 64.5°S, 64.5°W, near Palmer Station. Statistical analyses We used Pearson’s R correlation and linear regression tests (StatPlus:Mac) to determine relationship direction (positive or negative) and significance between climate indices and physical and biological parameters. Stepwise regression We conducted a stepwise regression analysis in MATLAB for both Palmer Stations B and E to determine the effects of both local (that is, wind, sea ice and water column stability) and large-scale (that is, SAM and MEI) physical forcing on the mean integrated, summer chl- a from both stations ( Fig. 3 ). Multiple model types were analysed that included many types of General Linear Models (GLMs) and the stepwise iterations added and removed individual model terms (for example, with or without monthly wind speed). Integrated chl- a at these two stations is not normally distributed; thus, we log transformed each chl- a value before performing the stepwise regression (and other analyses described above). Using GLMs requires that the dependent variable being modelled (in this case, chl- a ) must be normally distributed. After log transforming chl- a at each station, we used three different tests to determine whether the transformed data was from a normal distribution. These tests were Jarque–Bera [54] , Lilliefors [60] and χ 2 -goodness-of-fit using a 95% confidence interval. All three tests confirmed that the time series of log-transformed chl- a (dependent variable) from each station were from a normal distribution. In addition, to confirm that the linear relationships between the predictor variables and chl- a were not influenced by outliers in the predictor variables, we applied these same three tests of normal distribution to the residuals between modelled and observed chl- a . These tests confirmed that the residuals at both stations were from a normal distribution and thus were not influenced by outliers or highly skewed predictor variables. Finally, to determine whether the residuals between modelled and observed chl- a were autocorrelated (serial correlation) or not, we used the Durbin–Watson (dw) test [61] at a 95% confidence interval. The residuals of the model fits at both stations were not autocorrelated (Station B: dw=2.1288, P =0.8241; Station E: dw=1.6928, P =0.2532). Model selection was based on the corrected Akaike Information Criterion [62] (AIC c ). This information criterion selects the best model that simulates the observed data while taking into account both the sample size of the data set and the number of estimated parameters in each model. We tested a subset of non-linear models, and the linear models produced lower AIC c values with fewer predictor variables. The AIC c values for Stations B and E were −18.96 and −25.02, respectively. The regression was conducted using only the vertically integrated chl- a data from the summer months of December–January–February, which are the most consistent sampling months for the LTER time series. Therefore, we selected the model to simulate log mean monthly depth-integrated chl- a (mg chl- a m −2 ) from December–February. (log summer chl- a ; n =36 for Station B and n =38 for Station E). The highest ranked predictor variables for both Stations B and E summer chl- a were spring (September–October–November) SAM (SAM_SON), Δsigma-theta T min−0 _November/December (kg m −3 m −1 ), WAP August ice extent (km 2 ), wind threshold (number of days per season wind speeds were <2.5 m s −1 ) and various interactions between these variables. Statistics for each predictor are presented in Supplementary Table 1 . The GLMs used to simulate log summer chl- a (mg chl- a m −2 ) for Stations B and E are: Station B log summer chl- a =0.32287+(0.041656 × days per season under 2.5 m s −1 )+(0.0000063299 × WAP August ice extent)+(−96.913 × B_Δsigma-theta T min−0 _November/December)+(−0.28428 × SAM_SON)+(−0.00000011925 × WAP August ice extent × days per season under 2.5 m s −1 )+(1.938 × days per season under 2.5 m s −1 × B_ Δsigma-theta T min−0 _November/December)+(0.012671 × days per season under 2.5 m s −1 × SAM_SON)+(−19.88 × B_Δsigma-theta T min−0 _November/December × SAM_SON). Station E log summer chl- a =−2.5186+(0.12287 × days per season under 2.5 m s −1 )+(0.0000083066 × WAP August ice extent)+(−276.15 × E_Δsigma-theta T min−0 _November/December)+(−0.21811 × SAM_SON)+(−0.00000021796 × WAP August ice extent × days per season under 2.5 m s −1 )+(0.0070199 × SAM_SON × days per season under 2.5 m s −1 )+(0.00046018 × WAP August ice extent × E_Δsigma-theta T min−0 _November/December). Multicollinearity, a statistical phenomenon in which two or more predictor variables in a multiple regression model are highly correlated, can change parameter estimates, increase standard errors and reduce the power to detect reliable effects of correlated variables in the regression model [63] . To assess how much the variance of the coefficient estimate is being inflated by multicollinearity in our model, we determined the Variance Inflation Factors (VIFs) for each predictor variable used in the GLMs for Stations B and E chl- a . The typical rule of thumb is that multicollinearity can be ignored for a particular predictor variable if its VIF<4.0 (ref. 64 ). However, predictor variables that have a VIF of 4.0 or higher do not discount the regression analysis or call for the elimination of these predictor variables [64] . In our regressions, all VIFs were <4.0, which suggests that multicollinearity did not affect the GLM coefficient estimates or standard errors ( Supplementary Table 2 ). How to cite this article: Saba, G. K. et al . Winter and spring controls on the summer food web of the coastal West Antarctic Peninsula. Nat. Commun. 5:4318 doi: 10.1038/ncomms5318 (2014).